Retro-biosynthetic screening of a modular pathway design achieves selective route for microbial synthesis of 4-methyl-pentanol Increasingly complex metabolic pathways have been engineered by modifying natural pathways and establishing de novo pathways with enzymes from a variety of organisms. Here we apply retro-biosynthetic screening to a modular pathway design to identify a redox neutral, theoretically high yielding route to a branched C6 alcohol. Enzymes capable of converting natural E. coli metabolites into 4-methyl-pentanol (4MP) via coenzyme A (CoA)-dependent chemistry were taken from nine different organisms to form a ten-step de novo pathway. Selectivity for 4MP is enhanced through the use of key enzymes acting on acyl-CoA intermediates, a carboxylic acid reductase from Nocardia iowensis and an alcohol dehydrogenase from Leifsonia sp. strain S749. One implementation of the full pathway from glucose demonstrates selective carbon chain extension and acid reduction with 4MP constituting 81% (90±7 mg l −1 ) of the observed alcohol products. The highest observed 4MP titre is 192±23 mg l −1 . These results demonstrate the ability of modular pathway screening to facilitate de novo pathway engineering. Increasing interest in sustainable production of a wide range of chemical products has encouraged development of microbial catalysts for the conversion of renewable feedstocks to specialty and bulk chemicals as well as transportation fuels. Although natural hosts and metabolic pathways have been used for decades in the production of chemical products, the desire to synthesize direct replacements for current petroleum products has led to appropriation of natural pathways for production of noncognate chemicals [1] , [2] , [3] . Early examples of this new paradigm have focused on introducing or combining portions of natural pathways in alternative host organisms or creating new products by altering the termination of natural pathways of a host organism with promiscuous enzymes [1] , [3] , [4] , [5] , [6] , [7] , [8] , [9] , [10] , [11] . Recent work has been focused on improving modified natural pathways by substituting new enzymes to improve kinetics, improve expression or utilize alternate cofactors [12] , [13] , [14] . In some cases, pathways have been repurposed to synthesize new products by capitalizing on the natural capacity of enzymes to accept closely related substrates or by engineering protein specificity [15] , [16] , [17] . The boldest designs have utilized previously undescribed pathways created by combining the natural chemistry of individual enzymes from multiple hosts [18] , [19] , [20] . Liquid transportation fuels are one class of chemical targets for which natural pathways to exact replacements have not been discovered. Recent interest in microbial production of renewable fuels has led to successful synthesis of a variety of next-generation biofuels with improved properties over ethanol [12] , [14] , [15] , [21] , [22] , [23] , [24] , [25] , [26] , [27] . Microbial synthesis of these reduced chemical species by de novo designed pathways can potentially lead to more efficient production strains, which are necessary for next-generation targets to achieve commercial relevance. Predominantly, these pathways have employed reconstitution of natural pathways in new hosts (acetone-butanol-ethanol [5] , [6] ) or modified termination of natural pathways (fatty acid synthesis (FAS) [11] , [23] , [24] , amino acid synthesis [12] , [28] , isoprenoid synthesis [22] ). Although natural metabolites of lipid and terpene synthesis closely resemble biodiesel, there are few natural metabolites that closely mimic gasoline. Because gasoline constitutes 40% of total US petroleum consumption, a bio-based gasoline alternative would be useful for alleviating petroleum reliance. Two synergistic approaches are required for making a bio-based gasoline more economical: utilization of less expensive feedstocks and implementation of high-efficiency pathways [29] , [30] , [31] , [32] . The presented work focuses on development of a high-efficiency pathway for a bio-alternative alcohol for spark ignition engines. Such an alcohol would ideally fall in the C6–C7 range [25] , [26] , [33] . These medium-chain length alcohols achieve energy density equal to that of petroleum-derived gasoline (32 MJ l −1 ; Supplementary Fig. 1a ) [34] , [35] , [36] , [37] . Branched alcohols have the additional desired property of improved octane rating ( Supplementary Fig. 1b ) [33] . To date, the best examples of synthesizing such compounds have come from modified termination of branched amino-acid synthesis or from isoprenoid synthesis [22] , [28] . The amino acid-based pathway utilizes carbon chain extension by engineering α-ketoacid elongation (αKAE) enzymes and an α-ketoacid decarboxylase to produce a blend of alcohols. The inefficient carbon chain extension mechanism creates a redox imbalance for medium-chain products, which limits maximum pathway efficiency [38] . The isoprenoid pathway can be used to produce C5 isopentenol, but it is limited to forming carbon chain lengths in multiples of five because it uses isopentenyl diphosphate as a C5 building block, and it is limited by the inherent redox imbalance of the pathway. Here we present a pathway design, which combines a portion of a native pathway (valine biosynthesis) with a ten-step de novo pathway to produce 4-methyl-pentanol (4MP). To identify specific pathway variants, we utilize a conceptual modular framework based on general natural chemistries. Biosynthetic routes to alkyl chains most commonly employ a system of precursor generation followed by chain elongation through carbon–carbon bond-forming reactions [39] , [40] , [41] . We structure our conceptual modules to correspond to this pathway structure. We envision precursor generating modules (glycolysis and modules 1 and 2) and carbon chain elongation modules (module 3) coupled to alcohol terminating modules (module 4). This approach produces a pathway with enzymes selected from nine different metabolic contexts (organisms and/or pathways). We select four enzymes to act on their presumed cognate substrates and apply six to presumed noncognate substrates in the engineered pathway. The core module 3 pathway architecture is based on synthetic coenzyme A (CoA)-dependent chemistry first understood in the acetone-butanol-ethanol pathway of Clostridium acetobutylicum . This CoA-dependent architecture has several advantages compared with the αKAE and isoprenoid pathways described above. Biosynthetic CoA-dependent pathways typically utilize acetyl-CoA building blocks and extend carbon chains through condensation reactions without release of CO 2 . The potential for generation of two reducing equivalents per acetyl-CoA generated from glycolysis perfectly balances with those consumed for reduction to a primary alcohol product [15] , [42] . Indeed, the presented pathway achieves redox neutrality and a maximum theoretical yield of 0.67 mol 4MP per mole glucose (0.38 gg −1 , 100% maximum pathway energy efficiency). β-Oxidation chemistry has been used for synthesis of several straight-chain acids and alcohols [5] , [6] , [16] , [21] , [43] . Unlike these previous demonstrations of CoA-dependent pathways, here we present the expansion of potential products to branched alcohols of medium chain length using independently selected enzymes chosen to enhance specificity for our desired intermediates. 4MP pathway description The 4MP pathway design does not rely on the simple transfer of a single recombinant pathway; rather, it relies on a patchwork of enzymes from multiple organisms and multiple natural pathways ( Fig. 1 ). 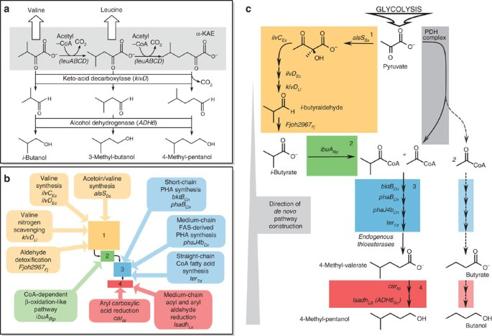Figure 1: 4-Methyl-pentanol (4MP) pathway schematic and alternative biofuel pathways. (a) The α-ketoacid elongation (αKAE) pathway was previously used to synthesize 4MP among other products. The αKAE route utilizes relatively inefficient single-carbon extension and non-specific decarboxylation and reduction of upstream precursors resulting in a redox imbalance and a mix of products, three of which are shown. (b) The presented CoA-dependent pathway to 4MP is assembled with genes from nine organisms taken from ten different pathway contexts. Pathway genes are shown with known native pathways or putative metabolic roles. Selectivity for 4MP was achieved while requiring enzymes for modules 3 and 4 to act on noncognate substrates. (c) The 4MP pathway can be organized into four modules, which were used to identify better performing enzymes for individual steps and validate portions of the overall pathway independentlyin vivo: Module 1, modified valine biosynthesis to isobutyrate; module 2, isobutyrate activation to isobutyryl-CoA; module 3, CoA-dependent condensation and reduction of isobutyryl-CoA and acetyl-CoA to 4-methyl-valerate (4MV); module 4, reduction of 4MV to 4MP. Genes in italics were overexpressed from plasmid sets. Modules were constructed working backwards from the 4MP product. A potential by-product shunt to butyrate and butanol was monitored during pathway construction. Figure 1 presents the overall pathway as a composite of four modules. Module 1, an adaptation of previously described routes to isobutanol and isobutyrate [12] , [44] , converts pyruvate, from glycolysis, to α-keto-isovalerate (α-KIV) via valine biosynthesis using Bacillus subtilis acetolactate synthase AlsS Bs , Escherichia coli acetohydroxy acid isomeroreductase IlvC Ec and E. coli dihydroxy acid dehydratase IlvD Ec . α-KIV is further converted to isobutyrate by the Lactococcus lactis decarboxylase KivD Ll and an isobutyraldehyde preferring aldehyde dehydrogenase from Flavobacterium johnsonaie (Fjoh_2967) [45] . Module 2 consists of the ATP-dependent activator Rhodopseudomonas palustris isobutyryl-CoA ligase IbuA Rp , which converts isobutyrate to isobutyryl-CoA [46] . Acetyl-CoA, generated by the endogenous pyruvate decarboxylase complex, condenses with isobutyryl-CoA in the first reaction of module 3, mediated by the Cupriavidus necator thiolase BktB Cn . The subsequent reactions of module 3 reduce the branched 3-keto-4-methylvaleryl-CoA intermediate to 4-methyl-valeryl-CoA by C. necator acetoacetyl-CoA reductase PhaB Cn , C. necator enoyl-CoA hydratase PhaJ4b Cn and Treponema denticola enoyl-CoA reductase Ter Td (refs 14 , 15 , 47 , 48 , 49 , 50 , 51 ). Endogenous thioesterase activity (potentially from TesB and YdiI [52] ) generates free 4-methyl-valerate (4MV). Module 4 reduces the free 4MV to 4MP by the Nocardia iowensis carboxylic acid reductase Car Ni and either Saccharomyces cerevisiae alcohol dehydrogenase Adh6p Sc or Leifsonia sp. strain S749 alcohol dehydrogenase Lsadh [53] , [54] , [55] , [56] , [57] (see Supplementary Fig. 2 for enzyme cofactor requirments and by-product reactions). Throughout this manuscript, strain names indicate the modules present in the strain (that is, M1F2I34 includes ‘M’ for modules, ‘1F’ for module 1 with feaB Ec , ‘2I’ for module 2 with ibuA Rp , ‘3’ for module 3 and ‘4’ for module 4). Strain names with ‘( )’ contain abbreviations for operon structure indicating the order of alsS Bs and ilvC Ec (that is, M1F(IA)2I34 includes (IA) indicating an ilvC Ec -alsS Bs operon order). 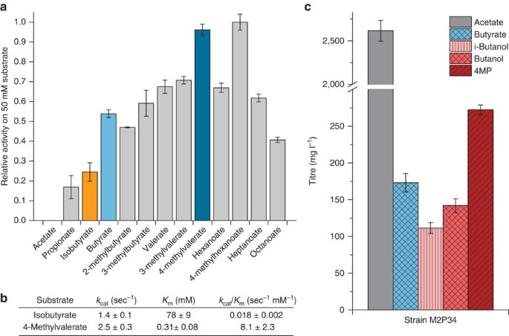Figure 2: Tuning of pathway selectivity by the carboxylic acid reductase CarNi. (a)In vitroanalysis of His-purified CarNireveals a dependence on acid primary-chain length with maximum activity at a chain length of five and six carbons. Branching at the C4 position is preferred significantly over straight acid species. The potential substrates for by-product formation, butyrate and isobutyrate, are seen to have 56% and 25% of the observed activity on 4-methyl-valerate (4MV), respectively. (b) Michaelis–Menten kinetics for isobutyrate and 4MV reveal that CarNihas a strong preference for the latter intermediate. (c) CarNisubstrate preference influences product selectivityin vivogenerating 1.9 times as much 4-methyl-pentanol (4MP; 272 mg l−1, 2.7 mM) as butanol (142 mg l−1, 1.9 mM) in strain M2P34 (expressing modules 2(pct), 3 and 4 genes) supplied with both glucose and isobutyrate. Even though 10 mM isobutyrate is supplied to the cultures of strain M2P34 only 111 mg l−1(1.5 mM) isobutanol is observed. All data are presented as the mean±s.d. (n=3) within vivodata generated using biological triplicates. See Table 1 and Supplementary Table 1 for descriptions of all strains used and Supplementary Table 2 for relevant descriptions of enzymes used in all pathway variants. Figure 1: 4-Methyl-pentanol (4MP) pathway schematic and alternative biofuel pathways. ( a ) The α-ketoacid elongation (αKAE) pathway was previously used to synthesize 4MP among other products. The αKAE route utilizes relatively inefficient single-carbon extension and non-specific decarboxylation and reduction of upstream precursors resulting in a redox imbalance and a mix of products, three of which are shown. ( b ) The presented CoA-dependent pathway to 4MP is assembled with genes from nine organisms taken from ten different pathway contexts. Pathway genes are shown with known native pathways or putative metabolic roles. Selectivity for 4MP was achieved while requiring enzymes for modules 3 and 4 to act on noncognate substrates. ( c ) The 4MP pathway can be organized into four modules, which were used to identify better performing enzymes for individual steps and validate portions of the overall pathway independently in vivo : Module 1, modified valine biosynthesis to isobutyrate; module 2, isobutyrate activation to isobutyryl-CoA; module 3, CoA-dependent condensation and reduction of isobutyryl-CoA and acetyl-CoA to 4-methyl-valerate (4MV); module 4, reduction of 4MV to 4MP. Genes in italics were overexpressed from plasmid sets. Modules were constructed working backwards from the 4MP product. A potential by-product shunt to butyrate and butanol was monitored during pathway construction. Full size image Table 1 Strains used for module and full pathway evaluation. Full size table Identification of acid and aldehyde reductases (module 4) Adoption of a CoA-dependent synthesis route required identification of pathways to link a saturated CoA thioester to the final alcohol product. The CoA thioester could be reduced by either a CoA-dependent aldehyde dehydrogenase or thioesterase/carboxylic acid reductase pairing. The resulting aldehyde could then be reduced by an alcohol dehydrogenase to generate the primary alcohol product. The wide array of identified alcohol dehydrogenases created a high probability that an alcohol dehydrogenase could be found for conversion to the final alcohol [13] , [58] , [59] . S. cerevisiae Adh6p Sc was initially selected because it was previously found to be a broad specificity alcohol dehydrogenase with high activity on medium- and branched-chain aliphatic aldehydes [53] . A smaller number of acid or CoA-thioester reductases have been characterized in the literature. From these previously identified enzymes, we looked to identify candidates with the potential to selectively convert 4MV to 4-methyl-valeraldehyde. Recently, a carboxylic acid reductase (Car) from Mycobacterium marinum was shown to convert a range of straight-chain fatty acids to fatty aldehydes, but with increasing catalytic efficiency ( k cat / K M ) for longer chain lengths [60] . A previously studied homologue, Car from N. iowensis , was found to have activity on a broad array of acids, but its activity on a range of aliphatic acids was not examined [61] . Car Ni from N. iowensis was selected for further study to determine whether it had specificity for targeted medium-chain branched acids. Assays were devised to confirm activity on desired substrates in vitro and in vivo . First, N-terminal His-tagged Car Ni was purified and assayed for relative activity on 13 straight and branched acid substrates from C2 to C8. Car Ni showed a peak in activity for acids with a primary chain-length of five or six carbons ( Fig. 2a ). The highest Car Ni activity was found for the branched species 4MV and 4-methyl-hexanoate. Given the need to reduce flux of precursors to undesired by-product alcohols, Car Ni was a logical selection because of its preference for 4MV over the short-chain acids acetate, isobutyrate and butyrate. A complementary in vivo assay was designed to examine the effectiveness of the module 4 pairing. Butyrate, valerate, 3-methyl-valerate, 4MV and hexanoate were fed to E. coli cultures expressing Car Ni /Adh6p Sc and conversion was monitored by sampling the culture media. OD 600 -normalized conversions followed a trend similar to observed in vitro results with maximal conversion for substrates with C5 primary chain length, as desired ( Supplementary Fig. 3 ). Figure 2: Tuning of pathway selectivity by the carboxylic acid reductase Car Ni . ( a ) In vitro analysis of His-purified Car Ni reveals a dependence on acid primary-chain length with maximum activity at a chain length of five and six carbons. Branching at the C4 position is preferred significantly over straight acid species. The potential substrates for by-product formation, butyrate and isobutyrate, are seen to have 56% and 25% of the observed activity on 4-methyl-valerate (4MV), respectively. ( b ) Michaelis–Menten kinetics for isobutyrate and 4MV reveal that Car Ni has a strong preference for the latter intermediate. ( c ) Car Ni substrate preference influences product selectivity in vivo generating 1.9 times as much 4-methyl-pentanol (4MP; 272 mg l −1 , 2.7 mM) as butanol (142 mg l −1 , 1.9 mM) in strain M2P34 (expressing modules 2(pct), 3 and 4 genes) supplied with both glucose and isobutyrate. Even though 10 mM isobutyrate is supplied to the cultures of strain M2P34 only 111 mg l −1 (1.5 mM) isobutanol is observed. All data are presented as the mean±s.d. ( n =3) with in vivo data generated using biological triplicates. Full size image Strong specificity of Car Ni for 4MV over isobutyrate was desired because isobutyrate is produced as an upstream intermediate. The Michaelis–Menten kinetic parameters of Car Ni were found using these two key intermediates to confirm the desired specificity ( Fig. 2b ). The k cat / K m ratio with 4MV was found to be 450 times higher than with isobutyrate, indicating the significant preference of Car Ni for 4MV over other acid substrates generated by the pathway. With a K m of 78±9 mM with isobutyrate, Car Ni is expected to convert isobutyrate poorly under physiologically relevant concentrations, which limits shunting of the precursor to isobutyraldehyde. Identification of dehydratases and reductases (module 3) Enzymes of the Clostridium acetobutylicum butanol pathway and enzymes from polyhydroxyalkanoate pathways have previously been used to synthesize straight chain butanol and pentanol [14] , [15] , [21] . Previous work from our group found the bktB Cn / phaB Cn combination is capable of synthesizing 3-hydroxy-4-methylvaleryl-CoA from isobutyryl-CoA and acetyl-CoA [50] . To the best of our knowledge, 3-hydroxy-acyl-CoA dehydratases and trans-enoyl reductases with activity on the subsequent branched intermediates have not been identified. From enzymes documented to have activity on straight medium-chain CoA substrates, 4 phaJ and 6 ter homologues were selected for further screening [48] , [49] ( Supplementary Table 1 ). An assay was developed to screen for enzymes with the desired activity by isolating modules 2 and 3 of our pathway in vivo with different combinations of dehydratases and reductases. Isobutyrate (10 mM) and glucose (1%) were supplied in lysogeny broth (LB) medium, and active gene combinations were identified by detecting 4MV secretion. The propionyl-CoA transferase from Megasphera elsdenii , pct Me , was used to activate isobutyrate [62] . Of the 24 combinations tested, phaJ4 homologues from Pseudomonas syringae, Pseudomonas aeruginosa and C. necator in combination with ter homologues from Vibrio parahaemolyticus and T. denticola produced 4MV ( Supplementary Fig. 4A ). The high producer, C. necator phaJ4b Cn / T. denticola ter Td (strain M3Sc-TdCn), yielded 297±45 mg l −1 4MV and was selected for module 3 moving forward. The previously used dehydratase hbd Ca and reductase crt Ca from the C. acetobutylicum butanol pathway were also tested in place of phaB Cn and phaJ4b Cn (strain M3Sc-Ca; Supplementary Fig. 4B ). Although some butyrate was produced by strain M3Sc-Ca, 4MV was not detected. With module 4 in vivo activity previously confirmed, 4MP production from glucose and isobutyrate was tested with a strain expressing modules 2, 3 and 4 genes (strain M2P34). As predicted by observed activities for Car Ni and Adh6p Sc , strain M2P34 preferentially produced 4MP (272±7 mg l −1 ) over isobutanol (111±7 mg l −1 ) and butanol (142±9 mg l −1 ) even while feeding 10 mM (870 mg l −1 ) isobutyrate ( Fig. 2c ). Glucose to isobutyryl-CoA (modules 1 and 2) Combining isobutyrate synthesis with CoA activation supplies the necessary isobutyryl-CoA precursor for 4MP synthesis from glucose or other simple carbon sources. The module 1 pathway was identified by building from the previous work of Zhang et al. , which synthesized isobutyrate in E. coli by combining valine biosynthesis with the L. lactis kivD Ll decarboxylase and various native aldehyde dehydrogenases, including PuuC and FeaB [44] . In previous work, our group has utilized the M. elsdenii transferase Pct Me for CoA activation of carboxylic acids including isobutyrate [50] . The ATP-dependent isobutyryl-CoA ligase (IbuA Rp ) from R. palustris provides an alternative activation mechanism for module 2, which creates a redox neutral overall pathway [46] . Multiple module combinations were used to explore the activities of the two E. coli aldehyde dehydrogenases selected for the final oxidation of isobutyraldehyde to isobutyrate. Module 1 expression with modules 2 ( pct Me ) and 3 led to the production of 4MV from glucose with titres up to 111±11 mg l −1 ( puuC Ec ) and 90±9 mg l −1 ( feaB Ec ; Supplementary Fig. 5A ). Module 1 with puuC Ec led to higher 4MV titres when coupled to modules 2 and 3, but it was possible that the E. coli aldehyde dehydrogenases had activity on the module 4 intermediate 4-methyl-valeraldehyde, which could regenerate 4MV and decrease reduction to 4MP when module 4 is added. Both aldehyde dehydrogenases were used for alternate versions of the full pathway, and only the feaB Ec strain (strain M1F2P34) produced 4MP (67±13 mg l −1 ), whereas the puuC Ec strain (strain M1P2P34) produced 4MV (67±11 mg l −1 ; Supplementary Fig. 5B ). In addition, the puuC Ec strain produced more butyrate (156±4 mg l −1 ) and less butanol (15±6 mg l −1 ) than the feaB Ec strain (62±15 mg l −1 butyrate, 49±17 mg l −1 butanol). Although a demonstration of 4MP synthesis from glucose was made, relatively low 4MP titres and high isobutyrate (1,113±34 mg l −1 ) and isobutanol (2,205±225 mg l −1 ) titres suggested there were possible bottlenecks in the initial strain, strain M1F2P34. The ATP-dependent isobutyrate activator, ibuA Rp , was used in place of the CoA transferase pct Me in order to relieve acetyl-CoA requirements and create redox neutrality for the pathway. New plasmid constructs were made to reorganize genes onto plasmids by module ( Supplementary Tables 1–3 ). It was anticipated that operon construction would reduce enzyme expression, especially for genes in the second position, but it was unknown if the effect would be detrimental to overall production without knowledge of the rate-limiting enzyme [63] . Two module 3 plasmid variants were tested to explore whether PhaB Re activity could become limiting when expressed from an operon used in the new constructs ( Supplementary Fig. 6A ). The variant with phaB Re in the first position of a two-gene operon generated higher titres supporting the theory that phaB Re could be the limiting activity within module 3. Comparison of phaB Cn expression from the two operon variants by SDS–polyacrylamide gel electrophoresis (SDS–PAGE) confirmed higher phaB Cn expression when placed in the first postion ( Supplementary Fig. 6B ). In addition, operon variants for alsS Bs and ilvC Ec expression were tested to examine if better balancing of flux between module 1 and the native acetyl-CoA pathway could improve 4MP production ( Supplementary Fig. 6A ). Placing alsS Bs in the second position while using the new plasmid constructs (strain M1F(IA)2I34) increased 4MP titres (168±31 mg l −1 ), whereas isobutyrate (290±24 mg l −1 ) and isobutanol (1,046±45 mg l −1 ) titres were reduced (see Supplementary Note 1 for further details). Based on available in vitro data and the presence of 4MV (42±7 mg l −1 ) even for improved strain M1F(IA)2I34, it was possible that FeaB Ec could be oxidizing 4-methyl-valeraldehyde into 4MV creating a futile cycle with Car Ni ( Fig. 3a , Supplementary Fig. 6C ). An aldehyde dehydrogenase Fjoh2967 Fj from F. johnsonaie had been found to prefer an isobutyraldehyde substrate over other aldehyde substrates when tested in vitro [45] . Replacing feaB Ec with Fjoh2967 Fj in strain M1Fj(IA)2I34 led to increased 4MP (193±23 mg l −1 , 0.033±0.005 mol mol −1 glucose) and elimination of detectable 4MV ( Fig. 3b ). Isobutyrate titres (424±9 mg l −1 , 0.084±0.004 mol mol −1 glucose) were increased and isobutanol titres (797±7 mg l −1 , 0.187±0.006 mol mol −1 glucose) were reduced ( Fig. 3c ). 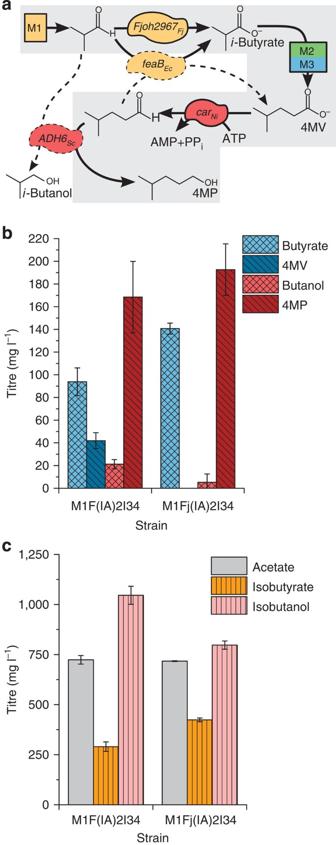Figure 3: 4MP synthesis from glucose improved through aldehyde dehydrogenase selection. (a) Key reactions involving aldehydes can generate futile cycles (aldehyde dehydrogenasefeaBEcwith the carboxylic acid reductasecarNi) or by-product shunts (alcohol dehydrogenaseADH6Sc). The desired pathway route is shown in bold arrows within the shaded box. Undesired reactions are shown with dashed arrows. Enzymes with insufficient selectivity have dashed outlines. (b) WhenfeaBEc(Strain M1F(IA)2I34) was replaced with the isobutyraldehyde-specific aldehyde dehydrogenaseFjoh2967Fjin strain M1Fj(IA)2I34 4MV titres were reduced and 4MP titres were increased. (c) Complementarily, strain M1Fj(IA)2I34 (Fjoh2967Fj) produced lower isobutanol and higher isobutyrate titres relative to strain M1F(IA)2I34 (feaBEc). All data are presented as the mean±s.d. (n=3) within vivodata generated using biological triplicates. Figure 3: 4MP synthesis from glucose improved through aldehyde dehydrogenase selection. ( a ) Key reactions involving aldehydes can generate futile cycles (aldehyde dehydrogenase feaB Ec with the carboxylic acid reductase car Ni ) or by-product shunts (alcohol dehydrogenase ADH6 Sc ). The desired pathway route is shown in bold arrows within the shaded box. Undesired reactions are shown with dashed arrows. Enzymes with insufficient selectivity have dashed outlines. ( b ) When feaB Ec (Strain M1F(IA)2I34) was replaced with the isobutyraldehyde-specific aldehyde dehydrogenase Fjoh2967 Fj in strain M1Fj(IA)2I34 4MV titres were reduced and 4MP titres were increased. ( c ) Complementarily, strain M1Fj(IA)2I34 ( Fjoh2967 Fj ) produced lower isobutanol and higher isobutyrate titres relative to strain M1F(IA)2I34 ( feaB Ec ). All data are presented as the mean±s.d. ( n =3) with in vivo data generated using biological triplicates. Full size image To examine if alcohol toxicity could be limiting product titres, toxicities of the dominant by-product isobutanol and desired product 4MP were assayed through exogenous addition of alcohols to the growth medium at concentrations from 1 to 10 mM. Isobutanol and 4MP concentrations up to 5 mM did not inhibit the exponential growth rate ( Supplementary Fig. 7 ). A combination of 10 mM (741 mg l −1 ) isobutanol and 2 mM (204 mg l −1 ) 4MP (comparable to titres observed for Strain M1Fj(IA)2I34) only reduced the exponential growth rate by 10%, the same reduction observed with 10 mM isobutanol alone. Although endogenously produced alcohols may be involved in alternative toxicity mechanisms, this result suggests that current titres are likely not limited by product toxicity. Pathway selectivity through enzyme selection (module 4) With knowledge of the specificity of Car Ni for 4MV over isobutyrate, the continued high isobutanol titres suggested Adh6p Sc was converting the isobutyraldehyde intermediate to isobutanol ( Fig. 4a ). Removing ADH6 Sc from Strain M1F(IA)2I34 produced strain M1F(IA)2I34a, which generated an isobutanol titre of 27±3 mg l −1 with nearly undetectable butanol and 4MP titres ( Fig. 4b ). An alternative to ADH6 Sc was identified from Leifsonia sp. strain S749. The new alcohol dehydrogenase Lsadh Ls was hypothesized to have improved specificity for 4-methyl-valeraldehyde based on substrates that were assayed in vitro [57] . When lsadh Ls was combined with the isobutyraldehyde-specific dehydrogenase Fjoh2967 Fj in strain M1Fj(IA)2I34L, selective synthesis of 4MP was achieved over other alcohol by-products ( Fig. 4c ). Isobutanol titres were reduced to 21±3 mg l −1 similar to those observed with the no alcohol dehydrogenase control. 4MP was produced at 90±7 mg l −1 (0.016±0.001 mol mol −1 glucose) making up 81% of all alcohol products. The dominant by-products were the 4MP precursors acetate (592±34 mg l −1 , 0.177±0.010 mol mol −1 glucose) and isobutyrate (1,128±34 mg l −1 , 0.229±0.002 mol mol −1 glucose), suggesting that by-product shunts were reduced and further improvement could be made by relieving a downstream rate limitation in modules 2, 3 or 4 ( Supplementary Fig. 8 ). Although 4MP titres were lower with Lsadh Ls , SDS–PAGE analysis of Lsadh Ls confirmed strong overexpression in E. coli ( Supplementary Fig. 8C ). The reduction in titre is likely due to the change from an NADPH-dependent dehydrogenase (Adh6p Sc ) to an NADH-dependent dehydrogenase (Lsadh Ls ) under the aerobic conditions used. The ratio of NADH/NAD + has been observed to be lower than that of NADPH/NAD + under similar culture conditions [64] . 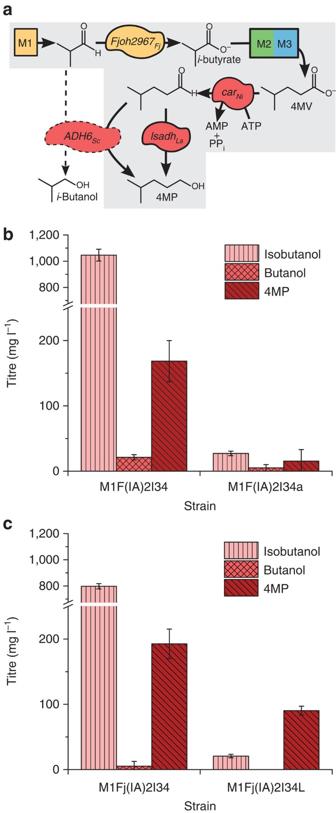Figure 4: Improved alcohol dehydrogenase selectivity withlsadhLs. (a) The desired pathway reactions to 4MP are indicated by bold arrows with the by-product shunt to isobutanol indicated by the dashed arrow. High activity of Adh6pScon isobutyraldehyde diverts isobutyrate flux to isobutanol. The LsadhLsalcohol dehydrogenase’s selectivity for 4-methyl-valeraldehyde greatly reduces flux to the isobutanol shunt. (b) The alcohol profile of strain M1F(IA)2I34 expressingfeaBEcandADH6Sccontains 168±31 mg l−1of 4MP but is dominated by 1.046±45 g l−1of isobutanol. The M1F(IA)2I34a control withoutADH6Scexpression produces low to undetectable levels of all three alcohols. (c) ReplacingfeaBEcwithFjoh2967Fjin strain M1Fj(IA)2I34 reduces isobutanol (797±20 mg l−1) and increases 4MP (192±23 mg l−1) marginally. ReplacingADH6ScwithlsadhLsgreatly enhanced alcohol selectivity producing 90±7 mg l−14MP with only 20±5 mg l−1isobutanol. All data are presented as the mean±s.d. (n=3) within vivodata generated using biological triplicates. Figure 4: Improved alcohol dehydrogenase selectivity with lsadh Ls . ( a ) The desired pathway reactions to 4MP are indicated by bold arrows with the by-product shunt to isobutanol indicated by the dashed arrow. High activity of Adh6p Sc on isobutyraldehyde diverts isobutyrate flux to isobutanol. The Lsadh Ls alcohol dehydrogenase’s selectivity for 4-methyl-valeraldehyde greatly reduces flux to the isobutanol shunt. ( b ) The alcohol profile of strain M1F(IA)2I34 expressing feaB Ec and ADH6 Sc contains 168±31 mg l −1 of 4MP but is dominated by 1.046±45 g l −1 of isobutanol. The M1F(IA)2I34a control without ADH6 Sc expression produces low to undetectable levels of all three alcohols. ( c ) Replacing feaB Ec with Fjoh2967 Fj in strain M1Fj(IA)2I34 reduces isobutanol (797±20 mg l −1 ) and increases 4MP (192±23 mg l −1 ) marginally. Replacing ADH6 Sc with lsadh Ls greatly enhanced alcohol selectivity producing 90±7 mg l −1 4MP with only 20±5 mg l −1 isobutanol. All data are presented as the mean±s.d. ( n =3) with in vivo data generated using biological triplicates. Full size image Recent efforts to develop microbial pathways for chemical synthesis have moved beyond upregulation of native pathways to include transfer and modification of heterologous pathways to new hosts and modified termination of native host pathways. Only a small number of truly de novo pathway designs have been published and most use isolated heterologous enzymes acting on their cognate substrates [18] , [19] , [20] , [50] . Engineered pathways to liquid fuels, in particular, have predominantly relied on entirely natural (ethanol, butanol, isoprenoid) or terminally modified natural pathways (FAS, amino-acid αKAE, isoprenoid). The presented work moves beyond modification of natural pathways by successfully demonstrating synthesis of a C6 branched alcohol via an extended de novo pathway, which maintains selectivity, while utilizing multiple naturally occurring enzymes outside their native pathway contexts. Although one set of modules has been presented in the current work, alternate chemistries could be substituted for or combined with the selected modules to create new pathways to the same or alternate products. For example, an isobutyryl-CoA mutase or branched α-keto-acid decarboxylase route could be used to generate the isobutyryl-CoA precursor in place of modules 1 and 2 (ref. 65 ). Similarly, a FAS route could be substituted for module 3 to generate the longer saturated acid substrate for module 4 (ref. 66 ). Using this design, individual alternative modules or module combinations can be directly compared with the existing pathway in vivo . In addition, entirely new classes of branched products (for example, aldehydes, alkanes) could be made by using different module 4 enzymes. For the presented pathway, an iterative screening approach identified the enzymes catalyzing conversion of the downstream 4-methyl-valeraldehyde and upstream isobutyraldehyde intermediates as key components controlling selectivity of the pathway. Our initial module 4 alcohol dehydrogenase selection, Adh6p Sc , proved to be highly active, but non-selective in the full pathway context. Module 4 displayed high activity on our desired substrate, but in vivo results with the full pathway suggested this module had a broad substrate range. Persistent high isobutanol titres from strains expressing modules 1–4 suggested that module 4 enzymes were interacting with isobutyrate and/or isobutyraldehyde. In vitro and in vivo data from module 4 testing implicated the alcohol dehydrogenase, Adh6p Sc , as the non-selective enzyme ( Figs 2 and 4 ). By replacing Adh6p Sc with the isobutyraldehyde-specific and NADH-dependent alcohol dehydrogenase, Lsadh Ls , pathway selectivity and overall cofactor utilization were improved. As with alcohol dehydrogenase candidates, we initially selected aldehyde dehydrogenases previously validated for an isobutyraldehyde substrate in an engineered pathway. Two endogenous enzymes, PuuC Ec and FeaB Ec , were previously identified as the most effective E. coli aldehyde dehydrogenases for isobutyraldehyde oxidation to isobutyrate [44] . Of the two E. coli aldehyde dehydrogenases, FeaB Ec proved to successfully synthesize 4MP from glucose in strain M1F2P34 expressing modules 1, 2, 3 and 4 ( Fig. 3b ). Based on in vitro data, one may predict PuuC Ec to function more effectively because its k cat / K m is more consistent across substrate lengths, whereas the k cat / K m of FeaB Ec actually increases by an order of magnitude between propionaldehyde and hexanaldehyde substrates [67] , [68] . In vivo results disproved this prediction with only FeaB Ec -producing 4MP ( Fig. 3a ). The better performance of FeaB Ec in the context of the full pathway may be explained by reported K m values for the two dehydrogenases. FeaB Ec has K m values below 100 μM for relevant substrates, whereas the K m values for PuuC Ec are 1 mM. PuuC Ec and FeaB Ec were tested in strains expressing ADH6 Sc . Like FeaB Ec , Adh6p Sc has reported K m values for relevant substrates in the 100–200 μM range [53] . Adh6p Sc was observed to have k cat values (~100 s −1 ) an order of magnitude higher than values observed for FeaB Ec and PuuC Ec (~10 s −1 ) for related aliphatic aldehydes. Together, these observed kinetics support the hypothesis that Adh6p Sc out-competes PuuC Ec and FeaB Ec for the isobutyraldehyde substrate. Isobutyraldehyde and reducing equivalents are diverted to isobutanol, lowering 4MP titres ( Supplementary Fig. 5 ). Strain M1P2P34 with PuuC Ec produces significantly more isobutanol than strain M1F2P34 with FeaB Ec , as expected based on observed K m values. In addition, in vitro data suggested that even though FeaB Ec functioned as an isobutyraldehyde dehydrogenase, it may also favour a 4-methyl-valeraldehyde substrate. The potential futile cycle created by activity on 4-methyl-valeraldehyde was avoided by using the isobutyraldehyde-specific dehydrogenase Fjoh2967 Fj from F. johnsonaie [45] . Replacing feaB Ec with Fjoh2967 Fj led to increased isobutyrate and eliminated detectable 4MV production ( Fig. 3 ). Combining more selective alcohol and aldehyde dehydrogenases led to a highly selective overall pathway with the major by-product being overflow of the upstream intermediate isobutyrate ( Supplementary Fig. 6 ). Together, the results from alcohol and aldehyde dehydrogenase selection highlight the importance of considering both high activity and required selectivity when utilizing retro-biosynthetic screening. Proposing potential upstream pathways is required to identify intermediates, which could have cross-reactivity with downstream enzymes. Further engineering of the CoA-dependent 4MP pathway is warranted given the potential high-energy yield. Dugar and Stephanopoulos have outlined the importance of balancing reducing equivalents generated and consumed in a recombinant pathway if high yields are desired [38] . Using the current 4MP pathway enzymes, the overall reaction can be written as: The reducing equivalents of the pathway are balanced, but some are contained in different cofactors. The maximum pathway energy efficiency ( γ P ) can be calculated using the degrees of reductance and pathway stoichiometry for a glucose substrate and 4MP product. Maximum pathway energy efficiency for the αKAE pathway and the presented CoA-dependent pathway are 75% and 100%, respectively. Accounting for cofactor requirements, the adjusted pathway energy efficiencies are 24% and 45% for the αKAE and CoA pathways, respectively ( Supplementary Methods ). If alternative enzymes are identified or engineered to accept NADH in place of NADPH, maximum pathway yields could be achieved under anaerobic fermentation. The maximum adjusted efficiency values for these pathway architectures then become 28% (αKAE) and 100% (CoA). The yield calculations highlight how our rational design approach leads to a pathway architecture with high-yield potential unlike inherently limited pathways utilizing modification of amino-acid synthesis. This work has identified a novel pathway for the selective synthesis of the branched medium-chain length alcohol 4MP. The highest titres (193±23 mg l −1 ) were achieved with strain M1Fj(IA)2I34, which expresses both Fjoh2967 Fj and ADH6 Sc . Selectivity was achieved by replacing ADH6 Sc with lsadh Ls in strain M1Fj(IA)2I34L. The 90±7 mg l −1 of 4MP produced by M1Fj(IA)2I34L represented 81% of observed alcohol products. In comparison, of the nine alcohols generated in the previous demonstration of microbial 4MP synthesis using α-KAE, 4MP (202.4±1.1 mg l −1 ) makes up 14% of the total alcohol product [28] . High potential efficiency and selectivity make our CoA pathway a preferred candidate for future engineering. Currently, the major by-products of the CoA-dependent route are the acids, acetate, isobutyrate and butyrate ( Supplementary Fig. 8 ). We expect that a combination of tuning thioesterase/transferase activities of the host to selectively cleave the longer 4-methyl-valeryl-CoA intermediate and relieving module 3 rate limitations will further enhance titres. Ultimately, screening or engineering for NADH-dependent enzymes should produce a high yielding fermentative pathway. Our existing pathway can also be adapted to produce other branched medium-chain products by testing new downstream modules. Finally, we believe the pathway design approach described here can be useful for creation of new metabolic pathways, which rely on long de novo routes. Retro-biosynthetic screening within a designed pathway framework enables exploration of enzymatic diversity using a small number of assays while preserving a maximally efficient biochemical conversion. Bacterial strains and plasmids E. coli MG1655(DE3) Δ endA ΔrecA described previously was the host strain for production experiments, alcohol toxicity experiments and for protein expression analysis using cell lysates [69] . E. coli DH10B (Invitrogen) and ElectroTen-Blue (Stratagene) were used in plasmid cloning transformations and for plasmid propagation. E. coli BL21Star(DE3) (Life Technologies) was used for expression of car Ni for purification (see Supplementary Tables 1 and 2 for strain details). A codon-optimized version of S. cerevisiae ADH6 was purchased from DNA 2.0 and codon-optimized versions of N. iowensis car and B. subtilis sfp were purchased from GenScript (see Supplementary Methods for codon-optimized sequences). Codon-optimized T. denticola ter and E. gracilis ter were purchased from GenScript [15] . Leifsonia sp. strain S749 lsadh was purchased as a codon-optimized GeneArt String from Life Technologies. All other genes were amplified from genomic DNA (gDNA). B. subtilis PY79, E. coli MG1655, P. putida KT2440, C. necator (formerly R. eutropha ) H16, M. elsdenii , R. palustris CGA009, P. syringae DC3000, C. acetobutylicum ATCC 824 and S. oneidensis MR-1 gDNA were prepared using the Wizard Genomic DNA purification Kit (Promega). P. aeruginosa PAO1-LAC (ATCC #47085), F. johnsonaie (ATCC #17061) and V. parahaemolyticus EB 101 (ATCC #17802) gDNA were purchased from American Type Culture Collection. Custom oligonucleotide primers were purchased (Sigma-Genosys) for PCR amplification of genes from gDNA using either Phusion High-Fidelity DNA polymerase (Finnzymes, Thermo Scientific Molecular Biology) or Q5 High-Fidelity DNA polymerase (New England Biolabs). Synthetic operons were constructed using a modified Splice by Overlap Extension PCR method. The compatible vector set pETDuet-1, pCDFDuet-1, pACYCDuet-1 and pCOLADuet-1 was used to express single genes or synthetic operons under control of a T7 lac promoter and individual ribosome-binding sites. Plasmids were constructed using standard molecular biology techniques with restriction enzymes and T4 DNA ligase purchased from New England Biolabs. Ligation products in pETDuet-1, pACYCDuet-1 and pCOLADuet-1 were used to transform E. coli DH10B and pCDFDuet-1 products were used to transform E. coli ElectroTen-Blue. Propagated constructs were purified using a QIAprep Miniprep Kit (Qiagen) and agarose gel fragments were purified using a Zymoclean Gel DNA Recovery Kit (Zymo Research). Completed constructs were used to co-transform E. coli MG1655(DE3) Δ endA Δ recA (see Supplementary Table 3 for plasmid details). Splice by overlap extension Initial PCR products with homologous ends were added to a PCR mixture without additional primers and cycled through a standard PCR cycle four times with annealing temperatures set at 6 °C above, 3 °C above and at the designed melting temperature for the homology. The upstream primer for the upstream gene and the downstream primer for the downstream gene in the designed operon were then added to amplify the full-length product. A standard PCR method using the annealing temperature for the primer pair was used for final amplification. Culture conditions For all production experiments, triplicate seed cultures were grown from isolated colonies at 30 °C overnight in 3 ml LB medium in a 14-ml culture tube on a rotary shaker at 250 r.p.m. All production cultures were inoculated with 1% inoculum from overnight seed culture and grown at 30 °C on a rotary shaker at 250 r.p.m. Cultures were induced with 0.5 mM isopropyl-β- D -thiogalactoside (IPTG) when OD 600 values reached 0.6–1.0 corresponding to mid-exponential phase. For constructs designed for 4MV production, 50 ml cultures in 250 ml shake flasks were used, and for constructs designed to produce 4MP, 3 ml cultures in 1 inch diameter 50 ml screw-cap culture tubes (Pyrex VISTA) were used. Unless otherwise stated, 1 ml culture samples were taken 48 h post induction, centrifuged to pellet cells, and the supernatant was removed for analysis. For production of 4MV and 4MP from glucose and isobutyrate, LB medium supplemented with 1% glucose and 10 mM isobutyrate was used. For production of 4MV and 4MP from glucose, LB medium supplemented with 1.2% glucose was used. Samples were taken 48 h post induction except for initial experiments with strains M1F2P34 and M1P2P34 when samples were taken 72 h post induction. For assessing toxicity of isobutanol and 4MP, an MG1655(DE3) Δ endA ΔrecA seed culture was grown overnight in LB medium. Duplicate 3 ml cultures in LB+1.2% glucose+alcohol were inoculated to an initial OD 600 of 0.1. Cultures were contained in the same 50 ml screw-cap tubes used in production experiments. Cultures contained 1 mM isobutanol, 5 mM isobutanol, 10 mM isobutanol, 1 mM 4MP, 5 mM 4MP, 10 mM 4MP or no alcohol. Growth was monitored by optical density and the growth rate was calculated from a linear regression of the natural log of the OD 600 values for the 1.5, 2 and 2.5 h post inoculation time points. Relative activity assay for purified His-Car An overnight culture of BL21 Star (DE3) (Invitrogen) harbouring pET/His-Car-RBS2-Sfp was used as 10% (v/v) inoculum in 2 l of LB broth. The culture was incubated at 30 °C and 250 r.p.m., and expression was induced using a final concentration of 1 mM IPTG at OD 0.6. Cells were harvested after 20 h using centrifugation and resuspended in a buffer containing 50 mM Tris-HCl pH 8.0, 300 mM NaCl and 10% glycerol. Cells were subsequently lysed using sonication. The supernatant was collected and applied to a column containing Ni-NTA resin (Qiagen). Affinity chromatography was performed using step-wise increasing concentrations of imidazole. Fractions containing purified His6-Car were dialyzed overnight at 4 °C into 50 mM Tris-HCl, pH 7.5, 50 mM NaCl, 1 mM DTT and 10% glycerol. Dialyzed enzyme was then flash frozen using liquid nitrogen and stored at −80 °C. The activity of His-Car on various substrates was determined by measuring changes in absorbance at 340 nm for up to 5 min in 96-well microplates (Tecan Infinite F200 Pro). Reactions were prepared as follows: 100 mM Tris-HCl, pH 7.5, 10 mM MgCl 2 , 0.6 mM NADPH, 1 mM ATP, 224 nM His-Car and 50 mM pH neutralized acid substrate. All substrates were assayed in triplicate. For K M and V max determinations, substrates were assayed at five different concentrations. SDS–PAGE analysis E. coli MG1655(DE3) Δ endA ΔrecA was transformed with empty pETDuet-1, pET-( bktB Cn -ter Td )-( phaB Cn -phaJ4b Cn ), pET-( bktB Cn -ter Td )-( phaJ4b Cn -phaB Cn ) pACYC-( car Ni -sfp Bs )- ADH6 Sc or pACYC-( car Ni -sfp Bs )- lsadh Ls . Single colonies from plates of each transformation were grown overnight in 3 ml of LB with appropriate antibiotic. Shake flask cultures (250 ml flasks) containing 50 ml LB+0.6% glucose were inoculated at 1% inoculum from overnight LB cultures and incubated with agitation at 30 °C and 250 r.p.m. Shake flasks were induced with 0.5 mM IPTG OD 600 values between 0.5 and 0.6. Five and a half hours after induction, 7 ml of each culture were sampled and pelleted by centrifugation. Cell pellets were resuspended in 1 ml of 10 mM Tris-HCl at pH 8.0 and added to 1.7 ml microcentrifuge tubes containing 500 μl of 0.1 mm diameter glass beads (Scientific Industries, Inc., Disruptor Beads, SI-BG01). Samples were then vortexed for 10 min. After lysis, samples were pelleted by centrifugation (6,000 g , 4 °C, 10 min) and the supernatant was removed as soluble lysate. Total protein was quantified by the Bradford assay method using Bio-Rad Protein Assay Dye Reagent (Bio-Rad, Cat #500-0006) and a bovine serum album standard [70] . A Bio-Rad 10% Mini-PROTEAN TGX gel (Bio-Rad, Cat #456-1034) was run using the Mini-PROTEAN Tetra Cell electrophoresis set up. Bio-Rad Precision Plus Protein All Blue Standard (Bio-Rad, Cat #161-0373) and 10 μg of total protein for each sample was loaded on the gel. After running at 200 V for 33 min, the gel was washed with deionized water before staining with Bio-Rad Bio-Safe Coomassie Stain (Bio-Rad, Cat #161-0786). Metabolite analysis Culture samples were pelleted by centrifugation and supernatant was removed for HPLC analysis with an Agilent 1,200 series instrument (Agilent) with a refractive index detector. Analytes were separated using the Aminex HPX-87H anion exchange column (Bio-Rad Laboratories) with a 5 mM sulfuric acid mobile phase at 35 °C and a flow rate of 0.6 ml min −1 . Commercial standards of glucose, α-KIV, acetate, acetoin, isobutyrate, butyrate, isobutanol, butanol, 4MV and 4MP were used for quantification of experimental samples by linear interpolation of external standard curves. How to cite this article : Sheppard, M. J. et al. Retro-biosynthetic screening of a modular pathway design achieves selective route for microbial synthesis of 4-methyl-pentanol. Nat. Commun. 5:5031 doi: 10.1038/ncomms6031 (2014).